Synthesis of chiral heterocycles by ligand-controlled regiodivergent and enantiospecific Suzuki Miyaura cross-coupling Non-aromatic nitrogen- and oxygen-containing heterocycles such as piperidines and pyrans are prevalent components of natural products and pharmaceutical drugs. Although it has been a workhorse as a synthetic method for assembling unsaturated sp 2 -hybridized substrates, transition metal-catalysed cross-coupling chemistry is traditionally not a suitable approach to prepare chiral non-aromatic heterocycles. Several mechanistic issues hamper the coupling of stereogenic secondary sp 3 -hybridized carbon-metal centres. Moreover, use of unsymmetrical allylic boronates in the Suzuki Miyaura cross-coupling is further complicated by the possibility of forming two regioisomeric products. Here we address this two-pronged problem and demonstrate that chiral enantiomerically enriched heterocyclic allylic boronates can be coupled with high stereochemical retention with a wide variety of aryl and alkenyl halides to independently afford both regioisomeric 2- and 4-substituted dihydropyrans and dehydropiperidines in high selectivity. A divergent mechanism is proposed where regiochemistry is governed by the nature of the ligands on the palladium catalyst. This scalable method is applied to the efficient preparation of the neuroactive alkaloid anabasine and the antidepressant drug paroxetine. Control of all levels of selectivity is essential to attain high overall efficiency when developing new reaction methods in organic synthesis. Chemoselectivity, the control of functional group reactivity, is a landmark achievement of modern transition metal-catalysed cross-coupling chemistry. The highly popular and Nobel prize-winning class of palladium-catalysed cross-coupling reactions achieves carbon–carbon bond formation between different functional groups with exquisite selectivity [1] . For example, in the highly popular Suzuki Miyaura cross-coupling reaction, the sp 2 -hybridized C–B bond of alkenyl or aryl boron compounds can be coupled selectively with the sp 2 -hybridized C–X bond of alkenyl or aryl halides ( Fig. 1a ) [2] , [3] , [4] , [5] . Coupling of sp 3 -hybridized partners such as alkylboron compounds is more challenging as it is rendered difficult by a slower transmetallation and possible side reactions such as β-hydride elimination [6] . When using chiral secondary alkylboron intermediates, these issues are compounded by the challenge of stereocontrol (control of the configuration of a stereogenic carbon). Indeed, although some progress has been realized in recent years [7] , [8] , [9] , [10] , [11] , [12] , [13] , [14] , [15] , [16] , [17] , [18] , [19] , [20] , control of stereoselectivity is viewed as one of the final frontiers in the Suzuki Miyaura reaction ( Fig. 1b ) [21] . With allylic boronates, the challenge of controlling selectivity is aggravated by the need to address a third type of selectivity arising from the possibility of forming two different regioisomers ( Fig. 1c ) [22] , [23] , [24] , [25] , [26] , [27] , [28] , [29] . Regioisoselectivity (or ‘site selectivity’) tends to be governed by the intrinsic steric and electronic effects dictated by the allylic substrate. When one of the two regioisomeric products forms favourably, it is notoriously difficult to invert this intrinsic preference. As such, it is challenging to develop reaction conditions that allow a divergent access to both regioisomers with high selectivity from a single substrate. Ultimately, the most desirable strategy is to employ catalysts as the controlling element. Organ [27] , then Yang and Buchwald [28] recently achieved this feat with a simple allylboronate devoid of stereochemistry. Crudden and co-workers [29] reported highly stereoretentive coupling with optically enriched acyclic allylboronates, however without controlling the formation of both regioisomers. 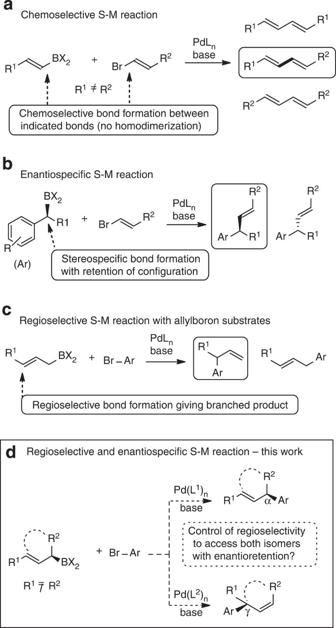Figure 1: Selectivity in Suzuki Miyaura (S–M) cross-coupling reactions. (a) A chemoselective S–M cross-coupling between two differently functionalized alkenyl (sp2hybridized) fragments, an alkenylboronic acid derivative and an alkenyl halide. (b) A stereospecific S–M cross-coupling where the configuration of the starting alkyl (sp3hybridized) boronate is preserved. (c) Cross-coupling of an unsymmetrical allylic boronate giving the branched product as favoured regioisomer. (d) The proposed and currently unaddressed merging of stereospecific and catalyst-controlled divergently regioselective cross-coupling to form both regioisomers independently. L, ligand. Figure 1: Selectivity in Suzuki Miyaura (S–M) cross-coupling reactions. ( a ) A chemoselective S–M cross-coupling between two differently functionalized alkenyl (sp 2 hybridized) fragments, an alkenylboronic acid derivative and an alkenyl halide. ( b ) A stereospecific S–M cross-coupling where the configuration of the starting alkyl (sp 3 hybridized) boronate is preserved. ( c ) Cross-coupling of an unsymmetrical allylic boronate giving the branched product as favoured regioisomer. ( d ) The proposed and currently unaddressed merging of stereospecific and catalyst-controlled divergently regioselective cross-coupling to form both regioisomers independently. L, ligand. Full size image In this article, we report a stereospecific Pd-catalysed Suzuki Miyaura reaction methodology where both regioisomer products of sp 2 –sp 3 cross-coupling reactions can be obtained independently with a remarkably high selectivity under the control of different ligands ( Fig. 1d ). By combining a full control of stereochemistry and regiochemistry, this cross-coupling process displays an unprecedented level of selectivity in the production of functionalized, chiral non-aromatic heterocycles such as piperidines and pyrans that possess great utility in the synthesis of natural products and pharmaceutical drugs [30] , [31] . In particular, this approach provides a new route to optically enriched 2- or 4-substituted arylpiperidines, which, in drug discovery, are deemed to be privileged compounds owing to the wide range of biological properties they are known to display (for example, 2-substituted: methylphenidate, mefloquine; 4-substituted: paroxetine, risperidone) [32] . Reaction design and preparation of substrates 3 and 4 The objective of preparing optically enriched 2- or 4-substituted pyran and piperidine derivatives by way of enantiospecific and regioselective allylic sp 2 –sp 3 cross-coupling methodology hinged on the preparation of suitable allylic boronate substrates. To realize this advance, we first developed a highly efficient catalytic enantioselective borylative isomerization of heterocyclic alkenyl triflates 1 and 2 ( Fig. 2 ). [33] , [34] The resulting chiral pyranyl and piperidyl allylic boronates 3 and 4 can lead to either α - or γ -regioselectivity in a Suzuki Miyaura cross-coupling with organohalide electrophiles (RX). This regioselectivity is tied to the mechanistic nature of the transmetallation step and whether it occurs with or without allylic rearrangement [22] , [23] , [24] , [25] , [26] , [27] . 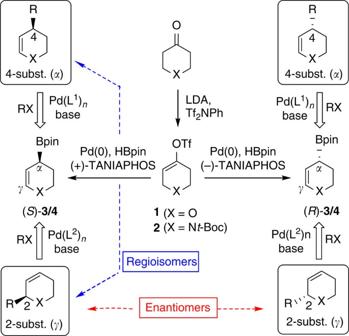Figure 2: Regioselective and enantiospecific S–M cross-coupling of heterocyclic allylic boronates3and4. By making use of antipodes of the chiral ligand TANIAPHOS in the catalytic enantioselective borylation of achiral enol triflates1and2, both enantiomers of3and4can be obtained in high selectivity. On a catalyst-controlled regiodivergent and stereospecific cross-coupling process, both 2- and 4-substituted regioisomeric products can be formed and isolated independently. The entire process thus lends access to all four possible isomeric piperidine and pyran isomers. Figure 2: Regioselective and enantiospecific S–M cross-coupling of heterocyclic allylic boronates 3 and 4 . By making use of antipodes of the chiral ligand TANIAPHOS in the catalytic enantioselective borylation of achiral enol triflates 1 and 2 , both enantiomers of 3 and 4 can be obtained in high selectivity. On a catalyst-controlled regiodivergent and stereospecific cross-coupling process, both 2- and 4-substituted regioisomeric products can be formed and isolated independently. The entire process thus lends access to all four possible isomeric piperidine and pyran isomers. Full size image Optimization and scope for dihydropyranyl boronate 3 Initial optimization of the regioselectivity was conducted on the racemic dihydropyranyl boronate 3 with 4-bromoanisole as the electrophile ( Table 1 ). At the onset, we planned to test out a variety of conditions and catalysts known to be particularly favourable for promoting Suzuki Miyaura cross-coupling reactions. Thus, strong σ -donor alkylphosphine ligands such as XPhos and tri- tert -butylphosphine were examined using different sources of palladium and bases. The use of [(allyl)PdCl] 2 , a Pd(II) complex precursor of Pd(0), and potassium phosphate in acetonitrile were shown to be essential (entries 1–6). In conjunction with XPhos as the ligand [4] , a high yield of 2-substituted coupling product 6 was obtained with exclusive γ -regioselectivity (entry 6). The effect of weaker σ -donating ligands on the regioselectivity was investigated, and although triphenylphosphine led to promising α -regioselectivity, product yield was low (entry 7). A re-examination of the reaction solvent identified acetonitrile as being optimal in affording a high yield of product (entry 10). When using tri(4-fluoromethylphenyl)phosphine, an excellent regioselectivity >17:1 was observed in favour of the α regioisomer 5 (entry 11). Use of Organ’s Pd-PEPPSI- i -Pr catalyst [27] , a N -heterocyclic carbene complex, afforded similar regioselectivity (entries 12 and 13). Table 1 Optimization of yield and regioselectivity in the Suzuki Miyaura coupling of dihydropyranyl boronate 3 . Full size table Optimization and scope for dehydropiperidyl boronate 4 Optimization of the cross-coupling between dehydropiperidyl boronate 4 and 4-bromoanisole is summarized in Table 2 . Application of the γ -selective conditions optimized for dihydropyran 3 was successful despite a lower yield (entry 1). A switch to potassium hydroxide as the base led to improved yields of 2-substituted dehydropiperidine 8 (entries 2 and 3). Preparation of the 4-substituted product 7 via an α -selective coupling was more challenging. The optimal conditions identified for dihydropyran 3 , using tris(4-fluoromethylphenyl)phosphine as the ligand, provided a moderate yield (entry 4). Switching to Pd-PEPPSI- i -Pr catalyst, however, afforded a significantly higher yield of product with excellent regioselectivity (entries 5 and 6). Contrary to the work of Organ and co-workers [27] , the corresponding i -Pent catalyst was less selective (entry 7). Table 2 Optimization of yield and regioselectivity in the Suzuki Miyaura coupling of dehydropiperidyl boronate 4 . Full size table A preliminary examination of the scope of suitable coupling partners for the optically enriched dihydropyranyl boronate 3 was performed ( Fig. 3 ). By applying the optimal conditions to favour the α coupling products using tris-4-trifluoromethylphenyl phosphine as a weak σ -donor ligand, aryl halides with both electron-donating and electron-withdrawing substituents as well as heteroaryl halides were successfully coupled in good to high yields to produce the 4-substituted regioisomers 5 and 9 – 15 with regioselectivity ratios ranging from 5:1 to 15:1. All regioisomers are separable by chromatography. It is remarkable that near or full retention of optical purity was observed for all of these examples. Even better regioisomeric control (over 98:2 ratio) was achieved under the γ coupling conditions for the formation of 2-substituted isomers 6 and 16 – 22 . As shown with the formation of 14 – 15 and 21 – 22 , both 1- and 2-substituted alkenyl halides are suitable electrophiles despite a lower regioselectivity under the γ -selective conditions. 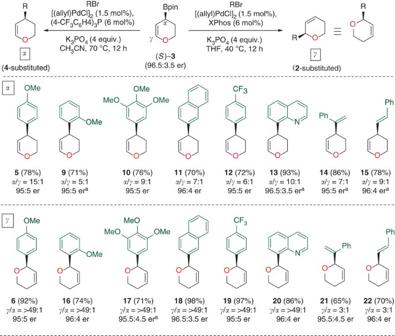Figure 3: Scope of electrophiles in the catalyst-controlled regiodivergent Suzuki Miyaura cross-coupling with dihydropyranyl boronate3. In the chemical equation on the top, variation of the R group in the electrophile under conditions of the left hand reaction provides viaαcoupling the 4-substituted dihydropyran products shown. Application of theγcoupling conditions on the right hand reaction provides the 2-substituted products. Below the structures of products, the isolated yield of the major, separated regioisomer is indicated in brackets next to the product number. Regioisomer ratio (α/γ) were measured from the1H NMR spectra of crude products, and, unless indicated otherwise,athe er’s were obtained directly from the pure coupling products by chiral HPLC analysis with a reasonable error of 2%. Note: reaction conditions and scale are indicated inTable 1and Methods. SeeTable 1for structure of XPhos.aer was measured after chemical derivatization as outlined in theSupplementary Information. Figure 3: Scope of electrophiles in the catalyst-controlled regiodivergent Suzuki Miyaura cross-coupling with dihydropyranyl boronate 3 . In the chemical equation on the top, variation of the R group in the electrophile under conditions of the left hand reaction provides via α coupling the 4-substituted dihydropyran products shown. Application of the γ coupling conditions on the right hand reaction provides the 2-substituted products. Below the structures of products, the isolated yield of the major, separated regioisomer is indicated in brackets next to the product number. Regioisomer ratio ( α / γ ) were measured from the 1 H NMR spectra of crude products, and, unless indicated otherwise, a the er’s were obtained directly from the pure coupling products by chiral HPLC analysis with a reasonable error of 2%. Note: reaction conditions and scale are indicated in Table 1 and Methods. See Table 1 for structure of XPhos. a er was measured after chemical derivatization as outlined in the Supplementary Information . Full size image Due to the importance of piperidines as a prominent class of saturated heterocycles in medicinal chemistry, we were pleased to observe a wide scope of aryl and alkenyl coupling partners for the piperidyl boronate 4 ( Fig. 4 ). Thus, the optimal conditions of Table 2 with Pd-PEPPSI- i Pr as catalyst for the α coupling provided the 4-substituted regioisomer with up to >98:2 selectivity. Starting from optically enriched boronate ( S )- 4 or ( R )- 4 with an optical purity of 97.5:2.5 enantiomeric ratio (er), coupling products 7 and 23 – 29 were all obtained with little or no erosion of enantiomeric purity with selectivities over 95:5 er. Selective γ coupling using XPhos as ligand was extremely effective, providing 2-substituted dehydropiperidines 8 and 30 – 36 in regioselectivities ranging from 15:1 to >98:2 and er’s over 95.5:4.5. In two cases ( 32 , 33 ), no erosion of enantiomeric purity was detected and coupled products were isolated with a 97.5:2.5 er. 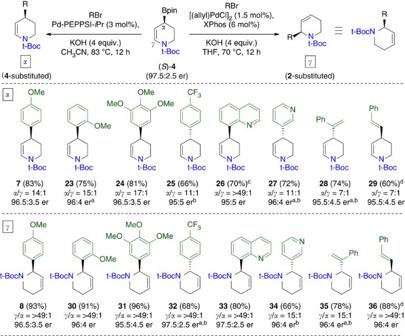Figure 4: Scope of electrophiles in the catalyst-controlled regiodivergent Suzuki Miyaura cross-coupling with dehydropiperidyl boronate4. In the chemical equation on the top, variation of the R group in the electrophile under conditions of the left hand reaction provides viaαcoupling the 4-substituted dehydropiperidine products shown. Application of theγcoupling conditions on the right hand reaction provides the 2-substituted products. Below the structures of products, the isolated yield of the major, separated regioisomer is indicated in brackets next to the product number. Regioisomer ratio (α/γ) was measured from the1H NMR spectra of crude products, and, unless indicated otherwise,athe er was obtained directly from the pure coupling products by chiral HPLC analysis with a reasonable error of 2%. Note. Reaction conditions and scale are indicated inTable 2and Methods. SeeTable 1for structure of Xphos and Pd-PEPPSI-i-Pr.aer was measured after chemical derivatization as outlined in theSupplementary Information.bProduct prepared from the enantiomeric substrate (R)-4.cTetrahydrofuran, 70 °C.dProduct prepared from a 4:1E/Zmixture of β-bromostyrene. TheEisomer reacts selectively and theZisomer is recovered unreacted.t-Boc, tert-butoxycarbonyl: (CH3)3COCO. Figure 4: Scope of electrophiles in the catalyst-controlled regiodivergent Suzuki Miyaura cross-coupling with dehydropiperidyl boronate 4 . In the chemical equation on the top, variation of the R group in the electrophile under conditions of the left hand reaction provides via α coupling the 4-substituted dehydropiperidine products shown. Application of the γ coupling conditions on the right hand reaction provides the 2-substituted products. Below the structures of products, the isolated yield of the major, separated regioisomer is indicated in brackets next to the product number. Regioisomer ratio ( α / γ ) was measured from the 1 H NMR spectra of crude products, and, unless indicated otherwise, a the er was obtained directly from the pure coupling products by chiral HPLC analysis with a reasonable error of 2%. Note. Reaction conditions and scale are indicated in Table 2 and Methods. See Table 1 for structure of Xphos and Pd-PEPPSI-i-Pr. a er was measured after chemical derivatization as outlined in the Supplementary Information . b Product prepared from the enantiomeric substrate ( R )-4. c Tetrahydrofuran, 70 °C. d Product prepared from a 4:1 E/Z mixture of β-bromostyrene. The E isomer reacts selectively and the Z isomer is recovered unreacted. t -Boc, tert-butoxycarbonyl: (CH 3 ) 3 COCO. Full size image Application to the synthesis of bioactive piperidines To demonstrate the practical usefulness of this methodology in the selective preparation of synthetic drug intermediates and natural products, we applied the regiodivergent piperidine couplings to the preparation of two neurologically active substances, ( S )-(+)-anabasine and (+)-paroxetine ( Fig. 5 ). To prepare ( S )-(+)-anabasine, a tobacco component formerly used as a botanical insecticide, piperidyl boronate ( R )- 4 was employed to prepare the γ coupling product 34 ( Fig. 4 ). The olefin of 34 was hydrogenated with diimide to provide the N -Boc-protected anabasine 37 in 95% yield without erosion of optical purity. Intermediate 37 can be transformed in a single high-yielding step to (+)-anabasine ( Fig. 5a ). 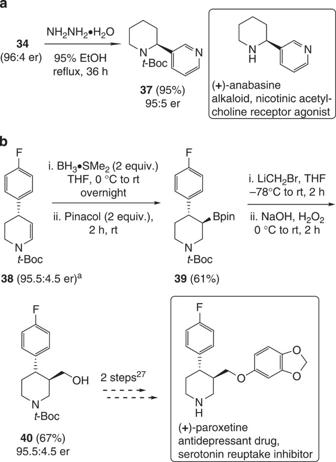Figure 5: Application of regiodivergent S–M cross-coupling products of heterocyclic allylic boronate4. (a) Formal synthesis of (+)-anabasine, a tobacco component and agonist of the nicotinic acetylcholine receptor. (b) Formal synthesis of (+)-paroxetine, a synthetic antidepressant drug of the selective serotonin reuptake inhibitor class.aProduct of a gram-scale reaction (with 1.4 g of (S)-4). [35] Figure 5: Application of regiodivergent S–M cross-coupling products of heterocyclic allylic boronate 4 . ( a ) Formal synthesis of (+)-anabasine, a tobacco component and agonist of the nicotinic acetylcholine receptor. ( b ) Formal synthesis of (+)-paroxetine, a synthetic antidepressant drug of the selective serotonin reuptake inhibitor class. a Product of a gram-scale reaction (with 1.4 g of ( S )-4). Full size image Paroxetine is a highly prescribed antidepressant drug belonging to the class of selective serotonin reuptake inhibitors. We accomplished a de novo catalytic enantioselective synthesis of ( 3S , 4R )-(+)-paroxetine from 4-aryl dehydropiperidine 38 , the product of a α -regioselective (α/ γ =11:1, separable) cross-coupling between boronate ( S )- 4 and 4-fluorophenyl bromide ( Fig. 5b ). This key coupling step was performed on a gram scale. The highly regio- and diastereoselective hydroboration [36] of 38 afforded secondary boronate 39 , which was subjected to a Matteson homologation [37] to afford, after an oxidative work-up, the alcohol intermediate 40 . Because the latter is a known, advanced intermediate to paroxetine [38] , this sequence constitutes a formal synthesis of (+)-paroxetine that can be accomplished in only seven steps from commercial t -Boc 4-piperidinone. This concise route compares favourably with the most recent enantioselective syntheses [39] , [40] , [41] , [42] , which were achieved, respectively, in 4 (82% ee) 8 (99% ee), 15 (95% ee) and 8 (94% ee) steps. The above-described syntheses of (+)-anabasine and (+)-paroxetine highlight how the use of a different catalyst/ligand in the Suzuki Miyaura cross-coupling provides a regiodivergent access to optically enriched piperidine derivatives of great utility in medicinal chemistry. Moreover, the residual unsaturation in the dehydro heterocyclic products offers numerous other opportunities to transform both the α and γ coupling products into more complex targets. Finally, by comparing with the known values of optical rotation, these syntheses confirmed the stereoretentive nature of these allylic cross-couplings. This cross-coupling methodology demonstrates an unprecedented level of regiochemical control with a near-perfect level of retention of stereochemistry. Three different catalyst–ligand systems have been identified to provide this level of control in the regiodivergent formation of α and γ regioisomers. As an attempt to rationalize these outcomes, Fig. 6a proposes a unifying mechanism for all three ligand systems: N -heterocyclic carbene (Pd-PEPPSI-iPr), XPhos and (4-CF 3 -C 6 H 4 ) 3 P. Under the aqueous base conditions employed, oxidative addition of the electrophile provides the hydroxyl-Pd(II) complex A. The ensuing transmetallation may occur through either an S E or S E ′ mechanism. The S E ′ mode of transmetallation is thought to be prevalent with phosphine-ligated Pd(II) species [25] , [29] . Thus, in these conditions, both XPhos and (4-CF 3 -C 6 H 4 ) 3 P are expected to first provide σ -bonded allylic Pd(II) complex B via a syn-S E ′ pathway made favourable through coordination of the electron-deficient Pd(II) to the electron-rich alkene. From complex B, the bulky strong σ -donor phosphine ligand XPhos provides the steric effect to encourage a prompt reductive elimination that yields the γ regioisomer product [4] , [28] , [43] . Being smaller and less conducive of reductive elimination, it is possible that the weaker, more labile σ -donor phosphine (4-CF 3 -C 6 H 4 ) 3 P encourages slippage of the η 1 σ -bonded complex B to the η 3 π-allyl intermediate C (that is, K σ - π >K RE ). The latter could now undergo π – σ equilibration between the two regioisomeric σ -bonded complexes B and D, which is presumed to favour D as the thermodynamic isomer due to heteroatom conjugation with the olefin [21] . Reductive elimination on complex D affords the α regioisomer. The NHC-ligated catalyst Pd-PEPPSI- i Pr appears to behave differently. This class of catalysts was previously alleged to transmetallate efficiently with simple allylboronic esters by a S E mechanism to give α substitution to the σ -bonded complex D directly [27] . This type of NHC complex is suspected to undergo a fast reductive elimination, and thus provide the α regioisomeric product with high selectivity. The reasons for its preference for a S E transmetallation are unclear, but it may be attributed to the bulk and non-dissociative character of the NHC ligand that disfavours an alkene-directed S E ′ mechanism. Because the C–B bond of A is ‘locked’ on a specific face of the allyl unit, the reaction is enantiospecific regardless of the three pathways described above. The observed retention of configuration is the outcome of a stereoretentive transmetallation followed by a stereoretentive reductive elimination [44] , [45] . Whereas the occurrence of enantiomeric erosion is possible in reactions of chiral π -allyl palladium complexes [46] , [47] , it is observed only to a minimal extent in these sp 3 –sp 2 cross-couplings. Although it requires supporting evidence, this mechanistic picture rationalizes the ligand-controlled regiodivergence in the formation of α and γ cross-coupling products and it highlights the important role of the heteroatom in providing a strong π -donating alkene that favors the S E ′ pathway when using XPhos or (4-CF 3 -C 6 H 4 ) 3 P as ligands, and in favouring the most stable σ -bonded Pd(II) complex D when using (4-CF 3 -C 6 H 4 ) 3 P. In contrast, the electronic properties of the alkene in heterocyclic allylboronates 3 and 4 should not play a determinant role when using the NHC ligand. Indeed, when using the carbocyclic analogue 41 , only Pd-PEPPSI- i Pr can promote the coupling to form 42 ( Fig. 6b ). 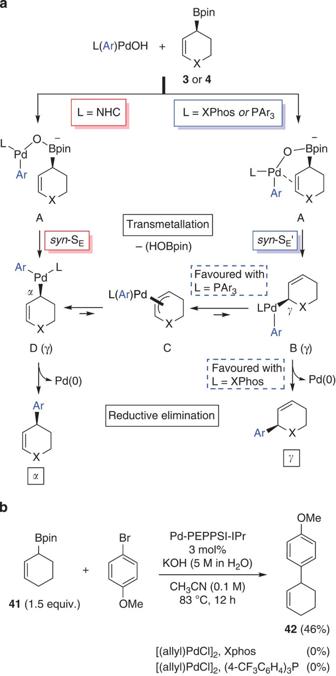Figure 6: Proposed mechanistic paths for the ligand-controlled regioselective S–M cross-coupling of heterocyclic allylic boronates3and4. (a) Use of different ligands leads to a mechanistic divergence where the NHC catalyst Pd-PEPPSI-iPr is alleged to promote a syn-SEtransmetallation and a fast reductive elimination to theαcoupling product (4-substituted). It is hypothesized that phosphine ligands XPhos and (4-CF3-C6H4)3P promote a syn-SE′ mechanism that can lead to both isomers depending on the rate of reductive elimination of intermediate B. Fast reductive elimination with XPhos (KRE>Kσ-π) leads to theγregioisomers, whereas slower reductive elimination with (4-CF3-C6H4)3P allows isomerization (Kσ-π>KRE) to the thermodynamically favouredσcomplex D affording theαcoupling product. (b) Control experiment showing that only the NHC catalyst Pd-PEPPSI-iPr is competent in the coupling with the non-heteroatom-conjugated allylboronate41, which supports the requirement for a strongπ-donating alkene as found in the heteroatom-conjugated substrates3and4, and a SE′ transmetallation with the phosphines XPhos and (4-CF3-C6H4)3P. Ar=(4-CF3-C6H4)3P. Figure 6: Proposed mechanistic paths for the ligand-controlled regioselective S–M cross-coupling of heterocyclic allylic boronates 3 and 4 . ( a ) Use of different ligands leads to a mechanistic divergence where the NHC catalyst Pd-PEPPSI- i Pr is alleged to promote a syn-S E transmetallation and a fast reductive elimination to the α coupling product (4-substituted). It is hypothesized that phosphine ligands XPhos and (4-CF 3 -C 6 H 4 ) 3 P promote a syn-S E ′ mechanism that can lead to both isomers depending on the rate of reductive elimination of intermediate B. Fast reductive elimination with XPhos (K RE >K σ - π ) leads to the γ regioisomers, whereas slower reductive elimination with (4-CF 3 -C 6 H 4 ) 3 P allows isomerization (K σ - π >K RE ) to the thermodynamically favoured σ complex D affording the α coupling product. ( b ) Control experiment showing that only the NHC catalyst Pd-PEPPSI- i Pr is competent in the coupling with the non-heteroatom-conjugated allylboronate 41 , which supports the requirement for a strong π -donating alkene as found in the heteroatom-conjugated substrates 3 and 4 , and a S E ′ transmetallation with the phosphines XPhos and (4-CF 3 -C 6 H 4 ) 3 P. Ar=(4-CF 3 -C 6 H 4 ) 3 P. Full size image In conclusion, this study demonstrates that a judicious choice of ligand for the palladium catalyst can successfully achieve a control of several levels of selectivity, notably, stereoselectivity and regioselectivity in the Suzuki Miyaura cross-coupling reaction. Such an ability to merge stereocontrol with a divergent control of regioselectivity was achieved with a class of heterocyclic substrates of tremendous importance in the field of drug discovery. This methodology provides a conceptually novel and general way of synthesizing optically enriched 2- and 4-aryl, -heteroaryl and -alkenyl piperidines and pyrans by direct sp 2 –sp 3 coupling. These findings provide much anticipation for the role of transition metal catalysis to greatly expand its breadth of application from its resounding success in the coupling of ‘flat’ sp 2 -hybridized substrates, to now include the construction of stereochemically defined sp 3 carbon centres in biologically relevant molecules with a potential for improved clinical success [48] , [49] . General considerations Reactions were performed under a nitrogen atmosphere using flame-dried glassware. Acetonitrile was distilled from CaH 2 . Tetrahydrofuran, toluene, dichloromethane and methanol were obtained from a MBraun MB SPS* solvent system before use. The anhydrous 1,4-dioxane was purchased from Sigma-Aldrich, 99.8%, and it was deoxygenated with dry nitrogen for 3 h before use. Pd(OAc) 2 was purchased from Sigma-Aldrich, ≥99.9%; chiral ligands (+)-TANIAPHOS and (−)-TANIAPHOS were synthesized on the gram scale, respectively, according to the literature procedure [50] . Other ligands and palladium catalysts were obtained from commercial sources. Thin layer chromatography was performed on Merck Silica Gel 60 F254 plates and was visualized with UV light and KMnO 4 stain. NMR spectra were recorded on Varian INOVA-300, INOVA-400 or INOVA-500 MHz instruments. The residual solvent protons ( 1 H) or the solvent carbons ( 13 C) were used as internal standards. 1 H NMR data is presented as follows: chemical shift in p.p.m. ( δ ) downfield from tetramethylsilane (multiplicity, coupling constant, integration). The following abbreviations are used in reporting NMR data: s, singlet; br s, broad singlet; d, doublet; t, triplet; q, quartet; dd, doublet of doublets; dq, doublet of quartets; qt, quartet of triplets, dtd, doublet of triplet of doublets; dse, double of septets; m, multiplet. High-resolution mass spectra were recorded by the University of Alberta mass spectrometry services laboratory using either electron impact or electrospray ionization techniques. Infrared spectra were obtained on a Nicolet Magna-IR with frequencies expressed in cm −1 . The enantiomeric excesses for chiral compounds were determined using a high-performance liquid chromatography (HPLC) Agilent instrument with Chiralcel-OD, IC, IB, or Chiralpak-AS columns. For 1 H and 13 C NMR analyses, see Supplementary Figs 1 to 84 . For HPLC analyses, see Supplementary Figs 85 to 159 . General procedure for examples of Figures 3 and 4 Complex [(allyl)PdCl] 2 (1.4 mg, 3.8 μmol) and ligand (15.0 μmol), or Pd-PEPPSI- i Pr (5.1 mg, 7.5 μmol) were added in a flamed-dried reaction tube, which was then flushed with nitrogen. The dry solvent (1.0 ml) was added and the mixture was stirred for 10 min. Heterocyclic allylboronic acid pinacol ester 3 (0.30 mmol, 1.2 equiv.) or 4 (0.38 mmol, 1.5 equiv.) was added via syringe, which was washed three times with dry tetrahydrofuran (0.5 ml portion). The aryl bromide (0.25 mmol) and aqueous base (1.25 mmol, 5 equiv.) were then added, and the resulting reaction mixture was allowed to stir under nitrogen at the designated temperature for 12 h. The mixture was allowed to cool down to room temperature, and passed though a short pipette loaded with silica gel, and rinsed with 15 ml of ethyl acetate. The solvents were then evaporated to yield a crude oil, which were subjected to flash chromatography (15% ethyl acetate/hexane) to afford the desired pyran or piperidine products. For detailed procedures and compound characterization data for compounds 5 to 40 , see Supplementary Methods . How to cite this article: Ding, J., Rybak, T. & Hall, D.G. Synthesis of chiral heterocycles by ligand-controlled regiodivergent and enantiospecific Suzuki Miyaura cross-coupling. Nat. Commun. 5:5474 doi: 10.1038/ncomms6474 (2014).